Enhanced ultra-low-frequency interlayer shear modes in folded graphene layers Few-layer graphene has attracted tremendous attention owing to its exceptional electronic properties inherited from single-layer graphene and new features led by introducing extra freedoms such as interlayer stacking sequences or rotations. Effectively probing interlayer shear modes are critical for unravelling mechanical and electrical properties of few-layer graphene and further developing its practical potential. Unfortunately, shear modes are extremely weak and almost fully blocked by a Rayleigh rejecter in Raman measurements. This greatly hinders investigations of shear modes in few-layer graphene. Here, we demonstrate enhancing of shear modes by properly folding few-layer graphene. As a direct benefit of the strong signal, enhancement mechanism, vibrational symmetry, anharmonicity and electron–phonon coupling of the shear modes are uncovered through studies of Raman mapping, polarization- and temperature-dependent Raman spectroscopy. This work complements Raman studies of graphene layers, and paves an efficient way to exploit low-frequency shear modes of few-layer graphene and other two-dimensional layered materials. Few-layer graphene (FLG) possesses unique properties of crystal structure, lattice dynamics and electronics. Rich physics and promising practical potential have been exploited, such as energy band gap opening in Bernal-stacked bilayer graphene (BLG) [1] ; varying responses in the integer quantum Hall effect measurements for ABA- and ABC-stacked trilayer graphene (TLG) [2] ; and the formation of Van Hove singularity (VHS) in folded or twisted double-layer graphene [3] , [4] , [5] , [6] . Raman spectroscopy is one of the most useful and versatile techniques to probe graphene layers as has been demonstrated in the studies of number of layers, strain, doping, edges, stacking orders, and even magneto–phonon coupling in graphene layers [7] , [8] , [9] , [10] , [11] , [12] , [13] , [14] , [15] , [16] , [17] , [18] , [19] , [20] , [21] , [22] . The unique and powerful advantage of Raman spectroscopy for probing graphene is the instant benefit of the truth that the fundamental vibrational modes such as G, G′ and D modes are highly involved in resonant scattering processes, which leads to a very strong signal, facilitates many unfulfillable measurements with a weak Raman signal and provides an effective way to probe phonons and electronic band structures through strong electron–phonon coupling (EPC). In addition to these well-known fundamental modes, some other weak modes such as higher order, combinational and superlattice wave vector-mediated phonon modes have been observed in either Bernal- or nonBernal-stacked graphene layers [23] , [24] , [25] , [26] , [27] , [28] . They all carry interesting and important information about lattice vibration and electronic band structures. Another very fundamental and intrinsic vibrational mode in FLG and bulk graphite is rigid interlayer shear mode, involving the relative motion of atoms in adjacent layers [29] , [30] . Vibrational energies of shear modes vary when the thickness and consequently the restoring force strength of Bernal-stacked graphene layers changes as being demonstrated by the experimental observation and perfectly modelled by a simple linear chin system [29] . Therefore, this shear mode, named C peak can be used as another Raman spectroscopic feature for identifying the thickness of Bernal-stacked graphene layers. Considering its low energy,~5 meV, researchers believe the C peak could be a probe for the quasiparticles near the Dirac point through quantum interference [29] . However, the low energy also causes direct observation of shear modes being extremely challenging, because the shear modes are so close to the excitation photons and fully suppressed by a notch or edge filter of most Raman instruments. To directly detect this C peak, low-doped Si substrate with pre-etched holes was used in the previous study [29] . Although the C peak of the suspended graphene layers was observed on such specially prepared substrate, it is still very weak, especially for BLG and TLG, which happen to be the most interesting and promising candidates of the graphene family together with single-layer graphene. Therefore, the extremely weak signal severely limits study of shear mode and its coupling with other particles. After the pioneering work [29] , very few experimental observations of the first-order fundamental shear modes of FLG were reported [31] . Here we report an enhancement of shear modes in folded graphene layers with certain rotational angles which also present the enhanced G mode due to the twist/folding induced VHS [32] . These folded graphene layers, including partially folded BLG, TLG and six-layer graphene are labelled as 2+2 r-f4LG, 3+3 r-f6LG and 6+6 r-f12LG, respectively, in this work. Here, ‘r’ refers to the enhanced G mode from the resonance scattering. Instead of specially prepared substrate of low-doped Si with array of micro-holes [29] , we use the typical substrates of highly doped Si with a 285-nm SiO 2 -capping layer. The extremely strong signal, comparable or even stronger than the enhanced G mode, enables measurements of two-dimensional (2D) Raman mapping, polarization- and temperature-dependent Raman spectroscopy of this low-frequency shear mode for the first time, and further unravels its enhancement mechanism, vibrational symmetry, anharmonicity and EPC. Enhanced shear modes by folding In our previous study, we classified folded graphene layers into three types by the folding or rotational angles θ as θ small , θ medium and θ large, for a given excitation laser. These three types of folded graphene layers exhibit very different Raman spectral features [32] . 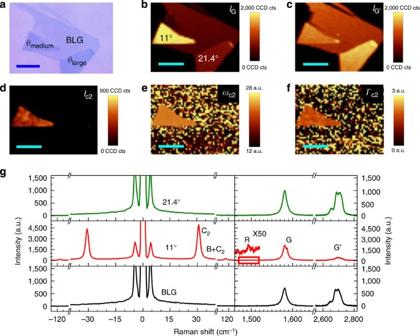Figure 1: Raman images and spectra of 2+2 f4LG. (a) Optical image of folded BLG. The folding types are identified and labelled by their rotational angles. (b,c) Raman intensity images of the G mode and G′ mode. (d–f) Raman image of intensity (d), frequency (e) and width (f) of the shear mode in 2+2 r-f4LG (C2). (g) Raman spectra of low and intermediate frequency modes of BLG,θmedium2+2 r-f4LG andθlarge2+2 f4LG. (Elaser=2.33 eV). Scale bars, 8 μm. Figure 1 shows BLG with two self-folded regions of rotational angles of 11° ( θ medium ) and 21.4° ( θ large, ). Excitation laser of 532 nm ( E laser =2.33 eV) was used for all the Raman measurements in this work. The significant enhancement of the G mode in the θ medium 2+2 r-f4LG can be clearly seen in the Raman image ( Fig. 1b ) and spectra ( Fig. 1g ). Surprisingly, along with the enhanced G mode, a low-frequency (~30 cm −1 ) peak also presents in this 2+2 r-f4LG, and it is so strong that the first Raman images of such low-frequency mode in graphene layers are clearly resolved by extracting its intensity, position and width ( Fig. 1d–f ). A single Lorentzian lineshape peak is used for fitting the Raman peaks in this study (see Supplementary Fig. 1 ). Reading the position and the width of this low-frequency mode and referring to the previous study of the suspended BLG [29] , we tentatively assign it to the interlayer shear mode (C peak or our label, C 2 ) of the ‘mother’ flake, BLG, but with an extremely large enhancement of the intensity. The good correlation between the enhanced C 2 and G modes is clearly revealed by the Raman images ( Fig. 1b,d ) and spectrum ( Fig. 1g ). Therefore, we believe that they share the same enhancement mechanism [4] , [6] . Although the formation and influence of VHS in folded or twisted 1+1 double-layer graphene has been intensively studied recently [3] , [4] , [6] , there is no evidence of the existence of such VHS in θ medium 2+2 r-f4LG. In this work, by adapting the previous methodology [33] , [34] , we exploit the electronic band structure and density of states of such 2D systems. The VHS with good corresponding to our excitation photon energy is seen (see Supplementary Fig. 2 ). We remark that the non-uniformity appearing in the Raman images of intensity of the C 2 mode ( Fig. 1d ) might be due to the varying of the interlayer spacing. A relatively weak peak locating at around 115 cm −1 is noticed and attributed to a combinational mode of interlayer breathing mode (~86 cm −1 ) [35] and the shear mode, labelled as B+C 2 peak herein. Figure 1: Raman images and spectra of 2+2 f4LG. ( a ) Optical image of folded BLG. The folding types are identified and labelled by their rotational angles. ( b , c ) Raman intensity images of the G mode and G′ mode. ( d – f ) Raman image of intensity ( d ), frequency ( e ) and width ( f ) of the shear mode in 2+2 r-f4LG (C 2 ). ( g ) Raman spectra of low and intermediate frequency modes of BLG, θ medium 2+2 r-f4LG and θ large 2+2 f4LG. ( E laser =2.33 eV). Scale bars, 8 μm. Full size image In addition to the enhancement of the G mode, unique Raman features such as ZO′, R and R' peaks mediated by either the short-range twisted bilayer lattice or the supperlattice have also been reported in 1+1 r-fDLG, and these modes exhibit obvious dependence of peak positions on twisting angles [25] , [36] . To further prove this newly observed ultra-strong low-frequency peak is the shear mode of the BLG and exploit its nature, we measured other two pieces of 2+2 r-f4LGs, which present R peaks of various positions ( Fig. 2 ). The rotational angles are determined by carefully fitting and reading the positions of R peaks [25] , [26] and double confirmed by both the optical and Raman images as previously reported [32] , [37] . Clearly enough, all C 2 peaks are enhanced and their positions show no dependence on the rotational angles, which is very much different to the twisting-angle-dependent peaks discussed previously. The detailed curve fitting and calculation (see Supplementary Table 1 ) show the peak positions and linewidths of these C 2 peaks, as well as the derived interlayer coupling strength by the frequencies of the C 2 peaks. The derived interlayer coupling strength keeps the same as that of normal Bernal-stacked BLG [29] . This indicates that the fundamental shear phonon mode of the ‘mother’ flake, although could be enhanced by the folding, is very robust even after being folded on top of itself, which must be very interesting and important for exploiting mechanical and electrical properties of such folded atomically thin layers including graphene and other 2D systems. It is also noticed that the position of the weak combinational (B+C 2 ) peak does not change when neither of the rotational angles vary. This further supports our assignment as both breathing (B) and shear (C 2 ) modes are the fundamental modes of the ‘mother’ flake and are not affected by the folding. 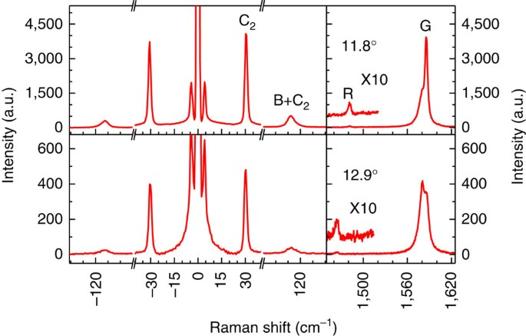Figure 2: Raman spectra of 2+2 r-f4LG. Raman spectra of low and intermediate frequency modes of 2+2 r-f4LG with different rotational angles as determined by the R peak positions and indicated. (Elaser=2.33 eV). Figure 2: Raman spectra of 2+2 r-f4LG. Raman spectra of low and intermediate frequency modes of 2+2 r-f4LG with different rotational angles as determined by the R peak positions and indicated. ( E laser =2.33 eV). Full size image Not only the 2+2 f4LG exhibits three types of folding, 3+3 f6LG also follows this criterion. 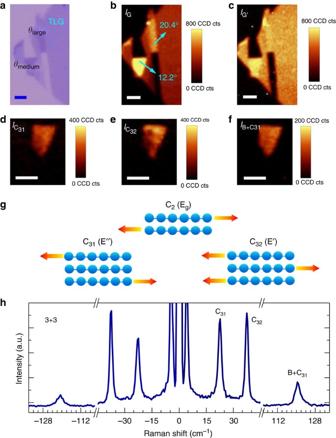Figure 3: Raman images and spectrum of 3+3 r-f6LG. (a) Optical image of folded TLG. The folding types are identified and labelled by their rotational angles. Raman intensity images of (b) G mode; (c) G′ mode; (d) lower-frequency shear mode (C31); (e) higher-frequency shear mode (C32) and (f) combinational mode (B+C31). (g) Schematic diagram of shear modes in BLG and TLG. (h) Raman spectrum of low-frequency modes of 3+3 r-f6LG with rotational angle of 12.2°. (Elaser=2.33 eV). Scale bars, 2 μm. Figure 3 presents optical and Raman images of θ medium and θ large 3+3 f6LG together with the Raman images of the low-frequency modes. The same as 2+2 r-f4LG, in the region of 3+3 r-f6LG, the low-frequency peaks are remarkably enhanced and correlate very well with the enhanced G mode as visualized by the Raman images. Therefore, the responsibility of the folding-induced VHS for the enhancement of G and C peaks could be extended to the 3+3 r-f6LG. As predicated by the theory [29] and illustrated by the diagram ( Fig. 3g ), there are two shear modes in Bernal-stacked TLG, locating at relatively lower- and higher-frequency sides of the shear mode in BLG. The Raman spectrum ( Fig. 3h ) of the 3+3 r-f6LG clearly presents two modes in the low-frequency region. The positions and linewidths (see Supplementary Table 2 ) guide us to assign these two modes as the Raman-active E″ shear mode for the lower-frequency one (C 31 ) and the infrared/Raman-active E′ shear mode for the higher-frequency one (C 32 ). Although C 31 is slightly weaker than C 32 , it is also significantly enhanced. This is the first observation of the lower-frequency shear mode, which is supposed to be extremely weak and could not be observed even in bulk graphite [29] . It is noticed that the interlayer coupling strength derived from the two shear modes of 3+3 r-f6LG is nearly identical to the one in the 2+2 r-f4LG and the previously reported [29] . The peak locating at ~120 cm −1 in the 3+3 r-f6LG is attributed to the combinational mode of the higher-frequency breathing mode (infrared-active) and the lower-frequency shear mode (Raman-active), labelled as B+C 31 . Very interestingly and meaningfully, in a 2+3-folded 5-layer graphene of a medium rotational angle (11.8°), G mode and shear modes of both BLG and TLG are enhanced (see Fig. 4 ). In a 6+6 r-f12LG, all five shear modes are clearly resolved and show perfect agreement with the theoretical predication (see Supplementary Fig. 3 ; Supplementary Table 3 ). This immediately indicates how robust the formation of VHS in such folded graphene layers, the enhancement of shear modes and G mode and the shear modes against the folding could be. The direct experimental observation of the entire set of the shear modes in folded FLG must be critical for future investigation of such interesting 2D systems. Figure 3: Raman images and spectrum of 3+3 r-f6LG. ( a ) Optical image of folded TLG. The folding types are identified and labelled by their rotational angles. Raman intensity images of ( b ) G mode; ( c ) G′ mode; ( d ) lower-frequency shear mode (C 31 ); ( e ) higher-frequency shear mode (C 32 ) and ( f ) combinational mode (B+C 31 ). ( g ) Schematic diagram of shear modes in BLG and TLG. ( h ) Raman spectrum of low-frequency modes of 3+3 r-f6LG with rotational angle of 12.2°. ( E laser =2.33 eV). Scale bars, 2 μm. 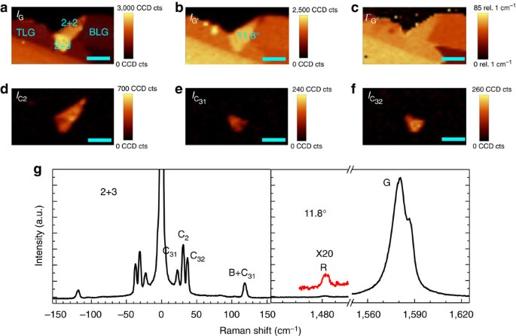Figure 4: Raman images and spectra of 2+3 r-f5LG. Raman image of (a) intensity of G mode; (b) intensity of G′ mode; (c) width of G′ mode. (d–f) Raman intensity images of shear modes in BLG (C2) and in TLG (C31and C32). (g) Raman spectrum of low- and intermediate-frequency modes of 2+3 r-f5LG. The shear modes of both BLG and TLG are enhanced together with the G mode. (Elaser=2.33 eV). Scale bars, 2 μm. Full size image Figure 4: Raman images and spectra of 2+3 r-f5LG. Raman image of ( a ) intensity of G mode; ( b ) intensity of G′ mode; ( c ) width of G′ mode. ( d – f ) Raman intensity images of shear modes in BLG (C 2 ) and in TLG (C 31 and C 32 ). ( g ) Raman spectrum of low- and intermediate-frequency modes of 2+3 r-f5LG. The shear modes of both BLG and TLG are enhanced together with the G mode. ( E laser =2.33 eV). Scale bars, 2 μm. Full size image Polarization dependence of enhanced shear modes Lattice vibrational symmetry, anharmonicity and EPC are some of the most important and fundamental properties of crystals, which are usually reflected by response of phonon modes to local disturbance. To further demonstrate the feasibility of the enhancement of shear modes by a proper folding and more importantly to exploit these intrinsic properties of FLG, we performed polarization and an in situ temperature-dependent Raman spectroscopy study. 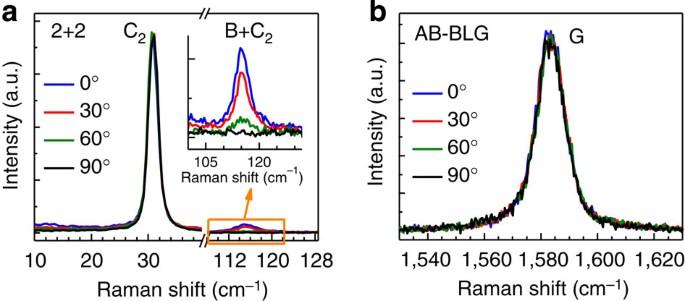Figure 5: Polarization-dependent Raman spectra of 2+2 r-f4LG. Raman spectra of (a) low-frequency modes and (b) G mode when the angles between the polarization of the incident and scattering lights are tuned to be 0°, 30°, 60° and 90° as indicated. (Elaser=2.33 eV). Figure 5 shows the low-frequency Raman modes and G modes of 2+2 r-f4LG as a function of angles between the polarization of the incident and scattering lights. The strong and sharp peak locating at ~30 cm −1 is inert to the change of polarization configurations, while the intensity of the weak peak locating at ~115 cm −1 is maximized under the parallel polarization and minimized for the perpendicular configuration. From our discussion and the assignments above, the enhanced sharp peak in the 2+2 r-f4LG should be the shear mode of Bernal-stacked BLG with the symmetry of E g . Thus, it is in-plane two-fold degenerated and naturally independent to our polarization configurations as G mode. For the weak peak, the assignment is the combinational modes of breathing (A 1g ) and shear ( E g ) modes in 2+2 r-f4LG. Since the out-of-plane breathing mode (A 1g ) contributes to the combinational modes, the intrinsic polarization nature of the A 1g mode is perfectly responsible for the polar dependence of the weak peaks locating at ~115 cm −1 , which shows zero intensity under anti-parallel and maximum for parallel polarization configuration. More discussion can be found in the Supplementary Information (see Supplementary Note 1 ). Figure 5: Polarization-dependent Raman spectra of 2+2 r-f4LG. Raman spectra of ( a ) low-frequency modes and ( b ) G mode when the angles between the polarization of the incident and scattering lights are tuned to be 0°, 30°, 60° and 90° as indicated. ( E laser =2.33 eV). Full size image Temperature dependence of enhanced shear modes In situ temperature-dependent Raman spectroscopy is one of the most powerful tools to probe phonons, an assembling of lattice vibration and their interaction with other particles/quasiparticles. In Fig. 6 , we present the evolution of the enhanced shear mode of BLG in a temperature range of 90–390 K. First, we compare our thermal chamber temperature readings with the sample local temperatures estimated from the intensity ratio of Stokes and anti-Stokes [38] (see Supplementary Note 2 ). The fairly good agreement between each other affirms that the laser heating could be neglected ( Fig. 6b ). Now, we focus on the line shift as a function of temperatures. A redshift of the shear mode as the increase of temperatures is observed ( Fig. 6c upper panel). In the previous studies, the similar redshift of the G mode is also reported, and the frequency of G mode at 0 K and the first-order temperature coefficient were extracted by a linear fitting [39] . Softening of phonons at a higher temperature is common for many crystals owing to the enlarged bonds length due to the thermal expansion. However, graphene is exceptional as it has quite a large negative thermal expansion, potentially leading to a blueshift instead, which actually has been well probed in the previous studies [40] , [41] . Although single-layer graphene anchoring on a substrate might be pinned down and follows the thermal expansion of the substrate, the shearing movement of the 2+2 f4LG should be much free. Thus, there must be extra contribution to the overall softening of the shear mode with the increase of temperatures. The response of phonon frequency to the temperatures is a very effective manifestation of the anharmonicity. Two effects are usually responsible for the temperature-dependent line shift: anharmonic multiple phonons coupling and crystal thermal expansion [40] . We speculate that the anharmonic multiple phonons coupling should be the main reason for the softening of shear mode phonons with the increase of temperatures. Following the previous strategy [40] , we fit our experimental data by a polynomial function, which carries the total effects of lattice thermal expansion and anharmonic phonons coupling. The perfect agreement of each other confirms our speculation. The frequency of the shear mode of BLG at 0 K is extrapolated to be ω (0)=32.6 cm −1 , which is critical for many further investigations, for example, probing the influence of phonon–phonon coupling on the linewidth of the phonon mode as discussed below. As comparison, the linear fitting is also shown here. Apparently, the nonlinear one is much more suitable, as also employed in the previous study [41] . 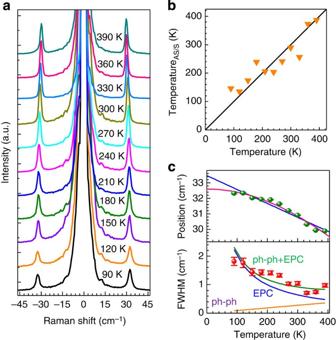Figure 6:In situtemperature-dependent Raman spectra of 2+2 r-f4LG. (a) Temperature-dependent Raman spectra of the shear mode with both Stokes and anti-Stokes lines. (b) Sample local temperatures estimated from the intensity ratio of Stokes and anti-Stokes as a function of the thermal chamber temperatures. (c) Positions (upper panel) and full width at half maximum (FWHM) (lower panel) of Stokes shear mode as a function of temperatures. The solid spheres represent the experimental data. The straight blue line (upper panel) is the linear fit and the pink curve is the polynomial fit, which accounts for both thermal expansion and anharmonic multi-phonon interaction. Obviously, the nonlinear fit is superior to the linear one. The frequency of the shear mode at 0 K can be extrapolated. For FWHM (lower panel), the green line is the fit of the data by considering both effects of the phonon–phonon (ph–ph) interaction and electron–phonon coupling (EPC). The purple and blue plots describe the contributions of the ph–ph and EPC, separately. The dominance of EPC, especially at low temperature is clear. Note: the FWHM has been corrected by subtracting the broadening of our system of 0.9 cm−1from the fitted values. The error bars shown here are s.e. of curve fitting. (Elaser=2.33 eV). Figure 6: In situ temperature-dependent Raman spectra of 2+2 r-f4LG. ( a ) Temperature-dependent Raman spectra of the shear mode with both Stokes and anti-Stokes lines. ( b ) Sample local temperatures estimated from the intensity ratio of Stokes and anti-Stokes as a function of the thermal chamber temperatures. ( c ) Positions (upper panel) and full width at half maximum (FWHM) (lower panel) of Stokes shear mode as a function of temperatures. The solid spheres represent the experimental data. The straight blue line (upper panel) is the linear fit and the pink curve is the polynomial fit, which accounts for both thermal expansion and anharmonic multi-phonon interaction. Obviously, the nonlinear fit is superior to the linear one. The frequency of the shear mode at 0 K can be extrapolated. For FWHM (lower panel), the green line is the fit of the data by considering both effects of the phonon–phonon (ph–ph) interaction and electron–phonon coupling (EPC). The purple and blue plots describe the contributions of the ph–ph and EPC, separately. The dominance of EPC, especially at low temperature is clear. Note: the FWHM has been corrected by subtracting the broadening of our system of 0.9 cm −1 from the fitted values. The error bars shown here are s.e. of curve fitting. ( E laser =2.33 eV). Full size image Now, we move to the linewidth. In a defect-free crystal, the intrinsic linewidth ( γ in ) is defined by: γ in = γ ph–ph + γ e–ph , where γ ph–ph represents the anharmonic phonon–phonon coupling and γ e–ph is from the electron–phonon interaction [42] . For γ ph–ph , a possible decay channel could be one shear mode phonon splits into two acoustic phonons of the same energy and opposite momentum [29] as described by: γ ph–ph = γ ph–ph (0)[1+2 n ( ω 0 /2)], where γ ph–ph (0) and ω 0 is the linewidth caused by the anharmonic phonon–phonon coupling and the frequency of the shear mode at 0 K, respectively. n ( ω T )=1/[exp( ħω T / K B T )−1] is the phonon occupation number, where ħω T is the shear mode phonon energy at temperature T and K B is the Boltzmann constant [43] . Rather than fixing the phonon energy, that is, 196 meV in the previous study of the G mode [40] , we substitute individual phonon energy of the shear mode at corresponding temperature because the variation of the G phonon energy is only around 0.3% in our temperature measurement window, whereas upto 8% is noticed for the shear mode phonon energy. EPC also contributes and even becomes a dominant contribution to linewidth in a gapless system such as graphene, graphite and metallic carbon nanotubes [15] , [44] . For γ e–ph , it should follow: γ e–ph = γ e–ph (0)[ f (− ħω /2 K B T )− f ( ħω /2 K B T )], where γ e–ph (0) is the width resulting from the EPC at 0 K and f ( x )=1/[exp( x )+1]. In this work, we fitted our data by considering both the anharmonic phonon decay ( γ ph–ph ) and the EPC ( γ e–ph ). A fairly good agreement could be achieved ( Fig. 6c ). γ ph–ph (0) and γ e–ph (0) are extrapolated to be 0.02 and 17.27 cm −1 , respectively. To further elucidate the origin of the linewidth or the phonon lifetime of the shear mode, we plot the contribution of γ ph–ph and γ e–ph in Fig. 6c . It is obvious that the γ e–ph is more dominant, especially at low temperatures. We expect a substantial EPC-induced increment of linewidth of shear mode at cryogenic temperature. Such decrease of phonon lifetime could be well interpreted as, at very low temperature the occupation of conduction band near the Dirac point by the thermal-excited electrons could be significantly suppressed, and as a result of the creation of phonon-excited electron–hole pairs and thus their interactions (EPC) are remarkably activated, leading to the broadening of Raman peaks. The large contrast of the phonon energies of the shear and G modes explains why the G mode is much broader than the shear mode, and a large EPC of the G mode could be preserved even at a high temperature [29] . Together with previous intensive Raman scattering studies of D, G and G′ modes of graphene layers, our systematic studies of the low-frequency interlayer shear modes of folded FLG complement the probing of fundamental Raman studies of layered carbon materials. The folding-induced VHS promotes a remarkable enhancement of the shear modes as it does on the G mode. The in-plane two-fold degenerated symmetry, the anharmonicity and EPC of the shear modes are well exploited through 2D Raman mapping, polarization- and temperature-dependent Raman spectroscopy of the strongly enhanced low-frequency shear modes in folded FLG (~5 meV), which was far away from being accessible before. More insight understandings of mechanical and electrical properties and further developments of practical applications of FLG are expected to be achieved soon through investigations of the enhanced shear modes in the stretched, electrically or molecularly doped folded FLG and even under a magnetic field. During the preparation of this manuscript, we became aware that the enhancement of shear modes in few-layer graphene scrolls was reported [45] . Sample preparation Graphene layers were prepared by the mechanical cleavage of graphite and transferred onto a 285-nm SiO 2 /Si substrate. During the mechanical exfoliation process, some graphene flakes flipped over and folded themselves partially and accidentally. Such interesting folded graphene layers were located under an optical microscope. The number of layers of the unfolded part was further identified by white-light contrast spectra and Raman spectroscopy [46] . The folding or rotational angles were determined by reading the R peak position [25] , [26] and double checked by their geometrical morphologies visualized in their optical and Raman images [37] . Raman spectroscopy study A WITec Raman system with a low-wavenumber coupler, a 600 lines per mm grating, a piezocrystal-controlled scanning stage, a × 100 objective lens of NA=0.95 was used for the Raman images. For Raman spectra, a 2,400 lines per mm grating was used and guaranteed a spectral resolution of 0.9 cm −1 , which was obtained by monitoring the linewidth of the Mercury atomic emission line. The in situ temperature-dependent Raman measurements were conducted in a Linkam thermal stage with a × 50-long working distance objective lens of NA=0.55. The linewidths of Raman peaks were corrected by subtracting the broadening of our system of 0.9 cm −1 from the fitted values. The s.e. of curve fitting were reflected by the error bars. All the Raman images and spectra were recorded under an excitation laser of 532 nm ( E laser =2.33 eV). To avoid the laser-induced heating, laser power was kept below 0.1 mW. How to cite this article: Cong, C. & Yu, T. Enhanced ultra-low-frequency interlayer shear modes in folded graphene layers. Nat. Commun. 5:4709 doi: 10.1038/ncomms5709 (2014).